Synergetic iridium and amine catalysis enables asymmetric [4+2] cycloadditions of vinyl aminoalcohols with carbonyls Catalytic asymmetric cycloadditions via transition-metal-containing dipolar intermediates are a powerful tool for synthesizing chiral heterocycles. However, within the field of palladium catalysis, compared with the well-developed normal electron-demand cycloadditions with electrophilic dipolarophiles, a general strategy for inverse electron-demand ones with nucleophilic dipolarophiles remains elusive, due to the inherent linear selectivity in the key palladium-catalyzed intermolecular allylations. Herein, based on the switched regioselectivity of iridium-catalyzed allylations, we achieved two asymmetric [4+2] cycloadditions of vinyl aminoalcohols with aldehydes and β,γ-unsaturated ketones through synergetic iridium and amine catalysis. The activation of vinyl aminoalcohols by iridium catalysts and carbonyls by amine catalysts provide a foundation for the subsequent asymmetric [4+2] cycloadditions of the resulting iridium-containing 1,4-dipoles and (di)enamine dipolarophiles. The former provides a straightforward route to a diverse set of enantio-enriched hydroquinolines bearing chiral quaternary stereocenters, and the later represent an enantio- and diastereodivergent synthesis of chiral hydroquinolines. Heterocycles are privileged motifs in fields ranging from pharmaceutical chemistry and agrochemistry to materials chemistry and life sciences. The development of efficient synthetic methods for preparing heterocyclic compounds has been a major focus of the synthetic community [1] , [2] . Among the continuing and productive efforts, catalytic asymmetric cycloadditions via transition metal (TM)-containing dipolar intermediates have been determined to be powerful tools for this purpose [3] , [4] , [5] . Within this realm of palladium catalysis, although many impressive advancements have been made regarding cycloadditions of Pd-containing dipolar intermediates with electrophilic dipolarophiles (Fig. 1a , path a: normal electron-demand cycloadditions) [6] , [7] , [8] , [9] , [10] , [11] , [12] , the inherent linear selectivity of Pd-catalyzed intermolecular allylic alkylation (AA) reactions renders the development of a general strategy for the coupling of such intermediates with nucleophilic dipolarophiles a formidable task (Fig. 1a , path b: inverse electron-demand cycloaddition) [13] , [14] . In the few known examples, some additional interaction (i.e., electrostatic interactions or hydrogen bonding interactions) between the Pd-containing dipole and nucleophilic dipolarophile was required to induce branched selectivity in the Pd-catalyzed intermolecular AA processes [15] , [16] , [17] , [18] , [19] . For this reason, the exploitation of alternative catalyst systems is required to develop general dipolar cycloadditions and efficiently utilize the synthetic potential of TM catalysis in the synthesis of heterocycles. Fig. 1 Research proposal on the Ir-catalyzed cycloadditions of vinyl aminoalcohols. a Well-developed dipolar cycloadditions through asymmetric palladium catalysis and remained problem. b Dipolar cycloadditions through asymmetric iridium catalysis Full size image Based on the pioneering works of Takeuchi [20] , [21] and Helmchen [22] , as well as the substantial contribution from Helmchen [23] , Hartwig [24] , Carreira [25] , You [26] and many other excellent scientists [27] , [28] , [29] , iridium-catalyzed AA reactions show excellent branched selectivity, which distinguishes them from Pd-catalyzed processes [30] . Recent studies have indicated that iridium catalysis is compatible with many other catalysis modes (i.e., phase catalysis [31] , amine catalysis [32] , [33] , [34] , Lewis base catalysis [35] , Brønsted acid catalysis [36] , and Lewis acid catalysis [37] , [38] , [39] , [40] ), significantly expanding the scope of Ir-catalyzed asymmetric allylic alkylation (AAA) reactions [41] . Inspired by these impressive achievements, we question whether a synergetic catalysis strategy involving iridium catalysis can be adopted to resolve the remaining problem associated with Pd-catalyzed inverse electron-demand cycloadditions. More interestingly, readily available vinyl aminoalcohols can be directly utilized as coupling partners in TM-catalyzed cycloadditions using Ir-containing dipoles (Fig. 1b ), avoiding the use of vinyl-substituted strained rings and carbonates like those required in Pd-catalyzed cycloaddition (Fig. 1a ). Here, through the combination of iridium and amine catalysis, we accomplished the [4+2] cycloadditions of vinyl aminoalcohols with aldehydes and β,γ-unsaturated ketones. Optically active quinolinones and tetrahydroquinolines were produced in good yields and with high diastereoselectivity and enantioselectivity. Design plan Hydroquinolines are a class of important aza-heterocycles that are ubiquitous in natural alkaloids and functional molecules (i.e., pharmaceuticals, agrochemicals, and chiral ligands) [42] , [43] , [44] . Among existing methods for synthesizing chiral hydroquinolines, catalytic asymmetric [4+2] cycloadditions stand out as one of the most streamlined approaches [45] , [46] , [47] , [48] , [49] . As part of our ongoing studies on the synthesis of heterocycles via TM-catalyzed cycloadditions [15] , [50] , [51] , [52] , [53] , [54] , [55] , in this work, we plan to develop reaction methodologies that utilize readily available reagents and feature good selectivity and high synthetic efficiency. A detailed description of a possible mechanism is outlined in Fig. 2 . We envision that two catalytic cycles could act in concert to realize this cycloaddition via the following steps: (1) the Ir catalyst reacts with vinyl aminoalcohol 1a to form Ir-containing dipole int. I [56] , [57] ; (2) the amine catalyst condenses with the aldehyde to generate enamine species II ; (3) these two transient species, I and II , react with each other to produce int. III , which can be further converted to hemiacetal 4 through an intramolecular cyclization ( III → IV ) and acid-promoted hydrolysis process ( IV → 4 ). Based on this mechanism, a diverse set of hydroquinolines can be generated in a facile manner by in situ conversion of the OH group to a variety of other functional groups ( 4 → 3 / 5 ). While attractive in theory, the construction of contiguous stereocenters and chiral all-carbon quaternary stereocenters [58] , [59] , [60] , [61] , [62] , as well as the compatibility between the catalysts, substrates, and additives are challenges that must be addressed. Fig. 2 Proposed mechanism. Synergetic iridium/amine catalysis for the enantioconvergent syntheses of hydroquinolines Full size image Condition optimization First, we investigated the Ir/amine-catalyzed cycloaddition/oxidation sequence using vinyl aminoalcohol 1a and aldehyde 2a . The use of 4 mol% of chiral Ir catalyst (2 mol% of [Ir(cod)Cl] 2 and 8 mol% of Carreira ligand L1 ) and 20 mol% of amine catalyst A1 , together with 0.5 eq. of CCl 3 CO 2 H and 1.0 eq. of H 2 O as additives, gave hemiaminal 4aa as a white solid in 92% yield; 4aa can be further oxidized to desired hydroquinone 3aa by PCC in 67% yield with 99% ee and >19:1 dr. The absolute configuration of product 3aa was determined by comparing the chiral HPLC spectra with a previous literature [55] . To circumvent the isolation of intermediate 4aa , we adopted an improved procedure that simply combined these two processes in one pot. 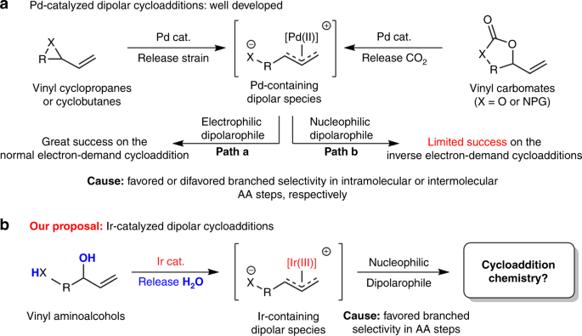Fig. 1 Research proposal on the Ir-catalyzed cycloadditions of vinyl aminoalcohols.aWell-developed dipolar cycloadditions through asymmetric palladium catalysis and remained problem.bDipolar cycloadditions through asymmetric iridium catalysis To our delight, quinolinone product 3aa was successfully generated with good reaction efficiency and excellent enantiocontrol under the standard conditions (Table 1 , entry 1: 64% yield, >99% ee and >19:1 dr). We then found that the protecting group on the nitrogen atom of the vinyl aminoalcohol had a substantial effect on the reaction selectivity. For example, when Boc-protected substrate 1a ′ was used instead of 1a , we only identified the byproduct from the allylation of CCl 3 CO 2 H (Table 1 , entry 2). It is worthy to note that, we have proven that the Ts group on product 3aa could be facilely removed by treatment with Mg powder in methanol (See Supplementary Procedure K). When vinyl aminoalcohol 1a ′′ was tested, there was almost no conversion of starting materials (Table 1 , entry 3). Furthermore, the effects of the acid and water as additives were investigated (Table 1 , entries 4–7). CCl 3 CO 2 H provided superior chemo- and enantioselectivities, and the addition of 1 eq. of water increased the reaction efficiency. Considering that the amine catalyst may play a key role in this reaction, various amine catalysts were examined. As shown in Table 1 , a bulkier amine, α,α-dimethyl benzylamine (Table 1 , entry 8, A2 ), gave only 22% yield, albeit with >19:1 dr and >99% ee. In addition, when chiral amine catalysts ( R )-A3 and ( S )-A3 were applied, we did not observe stereodivergent products, but the different amines did result in different reaction efficiencies (Table 1 entries 9 and 10). Table 1 Optimization of the reaction conditions for the [4+2] cycloaddition of vinyl aminoalcohols and aldehydes a Full size table Substrate scope Having established the optimal conditions, we started to explore the generality of the vinyl aminoalcohol substrate. 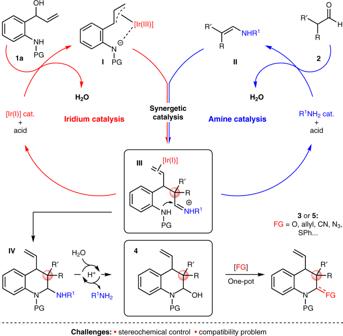Fig. 2 Proposed mechanism. Synergetic iridium/amine catalysis for the enantioconvergent syntheses of hydroquinolines As summarized in Table 2 , a wide range of vinyl aminoalcohols with electron-donating and electron-withdrawing groups, such as Me, F, and CF 3 , at the 5-position of the phenyl ring can readily react with aldehyde 2a to afford the desired dihydro-quinolinone products in moderate yields over two steps with high diastereo- and enantioselectivities (Table 2 , entries 1–4, 3aa – 3da : 59–66% yields, 6:1→ 19:1 dr and 94–99% ee). Furthermore, substrates with different substitution patterns, for example, 4-MeO, 4-Cl, and 6-F, were compatible with this asymmetric cycloaddition. The corresponding cycloadducts were achieved in satisfactory reaction efficiencies and stereoselectivities (Table 2 , entries 5–7, 3ea – 3ga : 61–73% yields, 12:1→19:1 dr and 98–99% ee). An allyl alcohol bearing a naphthyl moiety was also suitable for this reaction, and it was converted to product 3ha in 63% yield, 12:1 dr and 98% ee (Table 2 , entry 8). Table 2 Synthesis of Dihydroquinolinones form Various Vinyl Aminoalcohols a Full size table Subsequently, we explored an array of α-disubstituted aldehydes in this Ir- and amine-catalyzed cycloaddition/oxidation procedure. As summarized in Fig. 3 , the introduction of various groups at the para - or meta -positions of the 2-phenylpropanal was well tolerated in this reaction, and corresponding products 3ab – 3ai were obtained in good yields (55%−75% yields) and with high stereoselectivities (up to >19:1 dr and 96 → 99% ee). Moreover, aldehydes with naphthalene and other polycyclic systems can be converted to corresponding dihydro-quinolinones 3aj – 3am in good yields and excellent enantioselectivities (56–75% yields and up to >99% ee). Notably, an indole-derived substrate was also well tolerated in this reaction and provided a good result ( 3am , 56% yield, >19:1 dr and >99% ee). In addition, cyclic aldehydes with various ring sizes (i.e., five- or six-membered rings) could readily participate in this reaction ( 3an , 64% yield, >99% ee; 3ao , 74% yield, >99% ee). A dialkyl-substituted acetaldehyde, 2-methyl-3-phenylpropanal, could also be reacted under these conditions to give the desired product 3ap in a good yield and with an excellent enantioselectivity. A linear aldehyde, n -butanal, was also proven suitable for this transformation, affording dihydroquinolinone product 3ar in 31% yield, >99% ee and >20:1 dr (See Supplementary Procedure M). Fig. 3 Synthesis of dihydroquinolinones from various aldehydes. Reaction conditions: as indicated in entry 1 in Table 1 ; isolated yield; the ee and dr values were determined by chiral HPLC analysis Full size image Demonstrations of synthetic utility To illustrate the versatility of this cycloaddition, we explored various derivatizations of the hemiaminal intermediate. As highlighted in Fig. 4 , taking key hemiaminal 4aq (>99% ee and 5:1 dr), which was generated from the asymmetric cycloaddition of vinyl aminoalcohol 1a and isobutyraldehyde 2q , as an example, treatment with various organic reagents in one-pot reactions indeed provided a diverse set of functionalized hydroquinolines in generally high yields and excellent enantioselectivities. Except in the oxidation with PCC, the OH group of hemiaminal 4aq could be removed by treating the compound with Et 3 SiH and Et 2 O·BF 3 in DCM, giving tetrahydroquinoline 5b in 87% yield and >99% ee. Similarly, replacement of the hydroxyl group with other organosilicon reagents could deliver 2-allyl-, 2-CN- and 2-N 3 -substituted tetrahydroquinolines 5c – 5e in 84–91% yields and >99% ee, albeit with modest dr values. In addition, the OH group can be successfully converted to ether or sulfide moieties in good yields and excellent enantioselectivities ( 5f , 77% yield, 5:1 dr and >99% ee; 5 g , 76% yield, >19:1 dr and >99% ee. The high diastereoselectivity of product 5 g may be result of the steric effect (See Supplementary Procedures I and J), and its absolute configuration was established through the X-ray diffraction analysis (CCDC 1821791) [63] . Fig. 4 Divergent synthetic transformations of chiral hemiaminal 4aq . Reaction conditions: a ) PCC (5.0 eq. ), silica (100 mg), CH 2 Cl 2 (5 mL), 40 °C, 10 h; b ) Et 3 SiH (3.0 eq. ), Et 2 O·BF 3 (3.0 eq. ), CH 2 Cl 2 (3 mL), 0 °C, 5 min; c ) allyltrimethylsilane (3.0 eq. ), Et 2 O·BF 3 (3.0 eq. ), CH 2 Cl 2 (3 mL), 0 °C, 5 min; d ) TMSCN (2.0 eq. ), Et 2 O·BF 3 (3.0 eq. ), CH 2 Cl 2 (3 mL), 0 °C, 5 min; e ) TMSN 3 (2.0 eq. ), Et 2 O·BF 3 (3.0 eq. ), CH 2 Cl 2 (3 mL), 0 °C, 5 min; f ) p -TSA (20 mol%), EtOH (2.5 mL), 30 °C, 10 h. g ) PhSH (1.5 eq. ), Et 2 O·BF 3 (3.0 eq. ), CH 2 Cl 2 (3 mL), 0 °C, 5 min; isolated yield; the ee and dr values were determined by chiral HPLC analysis of purified products and 1 H NMR analysis of reaction mixtures, respectively. p -TSA: p -toluenesulfonic acid Full size image Stereodivergent [4+2] cycloadditions In addition to activating the α-position of the aldehyde via an enamine mechanism [64] , amine catalysis can also be used to efficiently activate the γ-position of the β,γ-unsaturated ketone through the formation of an dienamine species [65] , [66] , [67] , [68] , [69] . Based on this information and our above impressive results, we further probed the asymmetric [4 + 2] cycloadditions of vinyl aminoalcohols with β,γ-unsaturated ketones by merging iridium catalysis with dienamine catalysis. 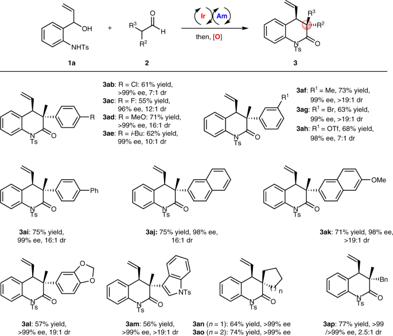Fig. 3 Synthesis of dihydroquinolinones from various aldehydes. Reaction conditions: as indicated in entry 1 in Table1; isolated yield; the ee and dr values were determined by chiral HPLC analysis With the cycloaddition of vinyl aminoalcohol 1a and ketone 6 as model substrates, a simple optimization of the reaction parameters including chiral amine catalyst, solvent, and acid defined the optimal reaction conditions (See Supplementary Table 3 for the details of condition optimization). To our delight, unlike the cycloaddition of vinyl aminoalcohols 1 with aldehyde 2 , which provides a pair of diastereomers, by reasonably using Carreira’s chiral phosphoramidite ligands, ( R )-L1 or ( S )-L1 , and Luo’s primary amine catalyst ( S )-A4 [70] , this reaction can provide both members of either of two pairs of diastereomers in good yields and with excellent enantio- and diastereoselectivities (Fig. 5 , ( R , R )- 7a , 84% yield, >99% ee and >19:1 dr; ( R , S )-7a , 81% yield, >99% ee and >19:1 dr). Worthy to note that, other two stereoisomers of 7a have been synthesized by using the enantiomer of Luo’s catalyst ( S )-A4 , too (See Supplementary Table 3 for details). The absolute configuration of product ( R , S ) - 7a were established by analyzing its derivative through the X-ray diffraction analysis (CCDC 1869868, See Supplementary Note 1 for details) [25] . Encouraged by these results, experiments to preliminarily examine the scope of vinyl aminoalcohols for this stereodivergent cycloaddition were performed. As highlighted in Fig. 4 , moderate to good yields together with high levels of enantio- and diastereocontrol were generally observed for both pairs of diastereomers. In a word, this is an interesting but challenging work that high diastereo- and enantioselectivities have been simultaneously accomplished in a stereodivergent manner, demonstrating the power and potential of synergetic catalysis strategies in the field of TM-catalyzed dipolar cycloaddition. Fig. 5 Enantioselective and diastereodivergent [4+2] cycloadditions of vinyl aminoalcohols and β,γ-unsaturated ketones. Reaction conditions: 1 (0.25 mmol), 6 (1.25 mmol), [Ir(cod)Cl] 2 (2 mol%), ( R )-L1 or ( S )-L1 (8 mol%), amine ( S )-A4 (20 mol%), in 1,2-dichloroethane (0.3 mL) for 48 h at 50 o C; isolated yield; the values of ee and dr were determined by chiral HPLC analysis Full size image Overall, we have successfully developed two enantioselective [4+2] cycloadditions of vinyl aminoalcohols with carbonyls, namely, aldehydes and β,γ-unsaturated ketones, through synergetic iridium and amine catalysis. The cycloaddition with aldehydes provides a diverse set of hydroquinolines bearing chiral quaternary stereocenters with a high level of enantiocontrol. 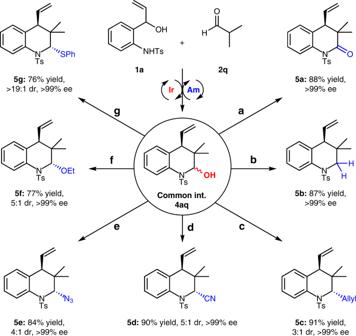Fig. 4 Divergent synthetic transformations of chiral hemiaminal4aq. Reaction conditions:a) PCC (5.0 eq.), silica (100 mg), CH2Cl2(5 mL), 40 °C, 10 h;b) Et3SiH (3.0 eq.), Et2O·BF3(3.0 eq.), CH2Cl2(3 mL), 0 °C, 5 min;c) allyltrimethylsilane (3.0 eq.), Et2O·BF3(3.0 eq.), CH2Cl2(3 mL), 0 °C, 5 min;d) TMSCN (2.0 eq.), Et2O·BF3(3.0 eq.), CH2Cl2(3 mL), 0 °C, 5 min;e) TMSN3(2.0 eq.), Et2O·BF3(3.0 eq.), CH2Cl2(3 mL), 0 °C, 5 min;f)p-TSA (20 mol%), EtOH (2.5 mL), 30 °C, 10 h.g) PhSH (1.5 eq.), Et2O·BF3(3.0 eq.), CH2Cl2(3 mL), 0 °C, 5 min; isolated yield; the ee and dr values were determined by chiral HPLC analysis of purified products and1H NMR analysis of reaction mixtures, respectively.p-TSA:p-toluenesulfonic acid 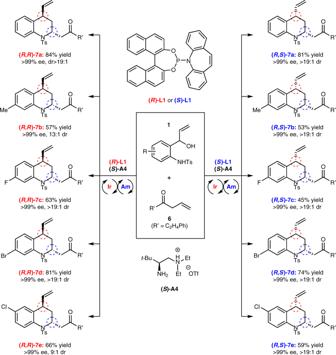Fig. 5 Enantioselective and diastereodivergent [4+2] cycloadditions of vinyl aminoalcohols and β,γ-unsaturated ketones. Reaction conditions:1(0.25 mmol),6(1.25 mmol), [Ir(cod)Cl]2(2 mol%),(R)-L1or(S)-L1(8 mol%), amine(S)-A4(20 mol%), in 1,2-dichloroethane (0.3 mL) for 48 h at 50oC; isolated yield; the values of ee and dr were determined by chiral HPLC analysis The reaction with β,γ-unsaturated ketones allows the enantio- and diastereodivergent synthesis of hydroquinoline products using reasonable chiral iridium catalysts and chiral amine catalysts. Obviously, the formation of Ir-containing dipoles from vinyl aminoalcohols and chiral iridium catalysts and (di)enamine dipolarophiles from carbonyls and amine catalysts provides a foundation for subsequent asymmetric [4+2] dipolar cycloadditions. As demonstrated in this work, the application of synergetic catalysis makes transition metal-catalyzed cycloadditions more practical and powerful for the synthesis of chiral heterocycles. Preparation of product 3 In a dried Schlenk tube under N 2 , [Ir(cod)Cl] 2 (0.005 mmol, 3.35 mg) and chiral ligand ( R ) - L1 (0.02 mmol, 10.15 mg) were mixed in 0.5 mL DCE and stirred at ambient temperature for 20 min under argon atmosphere. Then allylic alcohol 1 (0.25 mmol, 1.0 eq), aldehyde 2 (0.5 mmol, 2.0 eq), Cl 3 CCOOH (0.125 mmol, 20.4 mg), amine A1 (0.05 mmol, 9.2 mg, 8.7 μL), 4.5 μL H 2 O (1.0 eq.) were added to the mixture successively. The reaction mixture was stirred at ambient temperature until substrate 1 disappeared on TLC. Then the mixture was diluted with 5 mL DCM, PCC (275 mg, 5.0 eq.) and 100 mg silica gel were added to the mixture. The mixture was stirred at 40 o C for 12 h and the final product was achieved by flash column chromatography. Preparation of product 7 In a dried Schlenk tube under N 2 , [Ir(cod)Cl] 2 (0.005 mmol, 3.35 mg) and chiral ligand ( R )-L or ( S )-L1 (0.02 mmol, 10.15 mg) were mixed in 0.3 mL DCE and stirred at ambient temperature for 20 min under argon atmosphere. Then allylic alcohol 1 (0.25 mmol, 1.0 eq), ketone 2 (0.5 mmol, 2.0 eq) and chiral amine catalyst ( S )-A4 (0.05 mmol, 16.1 mg) were added to the mixture successively. After 8 h, the other 3.0 eq. ketone 2 was added in portions. Stirring at 50 o C for 48 h. The residue was directly purified by flash silica gel chromatography to afford the title compound.